Giant magnetic anisotropy and tunnelling of the magnetization in Li2(Li1−xFex)N Large magnetic anisotropy and coercivity are key properties of functional magnetic materials and are generally associated with rare earth elements. Here we show an extreme, uniaxial magnetic anisotropy and the emergence of magnetic hysteresis in Li 2 (Li 1− x Fe x )N. An extrapolated, magnetic anisotropy field of 220 T and a coercivity field of over 11 T at 2 K outperform all known hard ferromagnets and single-molecular magnets. Steps in the hysteresis loops and relaxation phenomena in striking similarity to single-molecular magnets are particularly pronounced for x ≪ 1 and indicate the presence of nanoscale magnetic centres. Quantum tunnelling, in the form of temperature-independent relaxation and coercivity, deviation from Arrhenius behaviour and blocking of the relaxation, dominates the magnetic properties up to 10 K. The simple crystal structure, the availability of large single crystals and the ability to vary the Fe concentration make Li 2 (Li 1− x Fe x )N an ideal model system to study macroscopic quantum effects at elevated temperatures and also a basis for novel functional magnetic materials. Controlling individual spins on an atomic level is one of the major goals of solid-state physics and chemistry. To this effect, single-molecule magnets (SMMs) [1] have brought significant insight ranging from fundamental quantum effects like tunnelling of the magnetization [2] and quantum decoherence [3] to possible applications in quantum computing [4] and high-density data storage [5] . Their basic magnetic units are coupled spins of a few magnetic atoms, which are embedded in and separated by complex organic structures. Whereas these are small magnetic units, they are still finite in extent and need to carefully balance coupling between magnetic atoms and isolation of one molecule from the next. Dimers of transition metals, as the small-size end point of SMMs, have been theoretically proposed to be promising candidates for novel information storage devices [6] . An alternative approach for the design of magnetic materials based on a few or even single atoms as magnetic units is ad-atoms on metallic surfaces [7] , [8] . The key property among these actually very different examples, and of any nanoscale magnetic system, is a large magnetic anisotropy energy. Basic magnetic units of SMMs are transition metal ion clusters [9] , lanthanide ion clusters [10] , [11] or mixed clusters of both [12] . Even mononuclear complexes based on a single lanthanide ion have been realized [13] , [14] . The lanthanide-based systems are promising due to their large single-ion anisotropy [15] , [16] , which often leads to large magnetic anisotropy energies. In contrast, single transition metal ions are seldom considered as suitable candidates and the number of reported attempts to use them as mononuclear magnetic units is limited [17] , [18] , [19] . The main reason is the widely known paradigm of ‘orbital quenching’. This suppression of the orbital contribution to the magnetic moment by the crystal electric field leads to a comparatively small anisotropy energy (neglecting spin-orbit coupling, a pure spin contribution is by default isotropic). The absence of an orbital contribution is reflected, for example, in the largely isotropic magnetization of the elemental ferromagnets Fe, Co and Ni [20] , [21] . However, Klatyk et al. [22] have suggested that a rare interplay of crystal electric field effects and spin-orbit coupling causes a large orbital contribution to the magnetic moment of Fe in polycrystalline Li 2 (Li 1– x Fe x )N. On the basis of the strong increase of the magnetization on cooling [22] and on Mössbauer spectroscopy [22] , [23] , a ferromagnetic ordering with T C ≈65 K was inferred for x =0.21 and, furthermore, huge hyperfine fields were found. The orbital contribution to the magnetic moment of Fe as well as the large hyperfine fields were theoretically described within the framework of local density approximation (LDA) calculations [22] , [24] . Furthermore, a large magnetic anisotropy has been theoretically proposed [22] , [24] . Here we show the experimental verification of the large anisotropy by magnetization measurements on single crystals and reveal a huge magnetic hysteresis as the key property of functional magnetic materials. More importantly, we have discovered that this highly anisotropic transition metal system manifests strong indications of a macroscopic quantum tunnelling of the magnetization in the form of pronounced steps in the magnetization loops and a temperature-independent relaxation. Tunnelling of the magnetization explicitly refers to the macroscopic tunnelling of the total magnetization and not to microscopic tunnelling events influencing the domain-wall movement in ferromagnets [25] . The Li 3 N host provides an extremely anisotropic ligand field for the Fe atoms as well as an insulating environment in analogy to the ‘organic framework’ of SMMs. There are no indications for meso- or macroscopic phase separation ( Supplementary Note 1 ). Although we cannot completely rule out cluster formation (for example, dimers or trimers of Fe on adjacent Li sites), the preponderance of the data supports a single iron atom as mononuclear magnetic centre, which is, furthermore, the simplest model and based on the fewest assumptions. The phenomenological similarities to SMMs indicate that the spontaneous magnetization and hysteresis are primarily caused by the extreme magnetic anisotropy and not by collective ordering phenomena. In accordance with earlier work on mononuclear systems, Li 2 (Li 1– x Fe x )N might be considered as ‘atomic magnet’ [26] or ‘single-ionic SMM’ [15] . The magnetic anisotropy, coercivity and energy barrier for spin inversion found in Li 2 (Li 1– x Fe x )N are roughly one order of magnitude larger than in typical SMMs. Magnetic hysteresis exists up to comparatively high temperatures of T ≳ 16 K for x ≪ 1 and is further enhanced up to T ≳ 50 K for the largest Fe concentration of x =0.28. Basic properties of Li 2 (Li 1– x Fe x )N We grew Li 2 (Li 1– x Fe x )N single crystals of several millimetre size ( Fig. 1a,b ) and Fe concentrations ranging over three orders of magnitude x =0.00028 to 0.28 by using a Li-flux method to create a rare, nitrogen-bearing metallic solution. Li 2 (Li 1– x Fe x )N crystallizes in a hexagonal lattice, space group P 6/ m m m , with a rather simple unit cell ( Fig. 1c ) and lattice parameters of a=3.652(8) Å and c=3.870(10) Å for x =0. Fe substitution causes an increase of a but a decrease of c by 1.1% and 1.5%, respectively, for x =0.28 with intermediate concentrations showing a linear dependence on x following Vegards law ( Supplementary Fig. 1 ). As indicated by the notation of the chemical formula, the substituted Fe atoms occupy only the Li-1 b Wyckoff position, which is sandwiched between Li 2 N layers. The iron concentrations, x , were measured by inductively coupled plasma mass spectrometry (ICP–MS), which enables a quantitative analysis on a parts per billion level ( Fig. 1d ). Structural parameters and selected x values were determined by single-crystal and powder X-ray diffraction and are in good agreement with earlier results [22] , [27] , [28] , [29] . To support our findings we present details of crystal growth procedure and chemical analysis (see Methods), as well as X-ray powder diffraction ( Supplementary Fig. 2 ; Supplementary Note 2 ) and X-ray single-crystal diffraction ( Supplementary Tables 1 and 2 ; Supplementary Note 3 ). 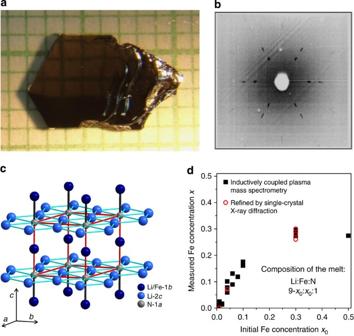Figure 1: Basic structural properties. (a) Single crystal of Li2(Li0.90Fe0.10)N on a millimetre grid and (b) corresponding Laue-back-reflection pattern. The crystal is not transparent and the faint grid pattern is a reflection off of the lens and the flat surface of the reflecting top facet. (c) Crystal structure with Li2N layers separated by a second Li site, which is partially occupied by Fe. The unit cell of the hexagonal lattice is indicated by red lines. (d) Measured Fe concentrationxas a function of the Fe concentration in the meltx0. For small concentrations,xtends to be larger thanx0, however, a plateau inxas a function ofx0emerges forx0≳0.3.xwas determined by both ICP–MS (see Methods) and refinement of single-crystal X-ray diffraction data (seeSupplementary Fig. 1). Figure 1: Basic structural properties. ( a ) Single crystal of Li 2 (Li 0.90 Fe 0.10 )N on a millimetre grid and ( b ) corresponding Laue-back-reflection pattern. The crystal is not transparent and the faint grid pattern is a reflection off of the lens and the flat surface of the reflecting top facet. ( c ) Crystal structure with Li 2 N layers separated by a second Li site, which is partially occupied by Fe. The unit cell of the hexagonal lattice is indicated by red lines. ( d ) Measured Fe concentration x as a function of the Fe concentration in the melt x 0 . For small concentrations, x tends to be larger than x 0 , however, a plateau in x as a function of x 0 emerges for x 0 ≳ 0.3. x was determined by both ICP–MS (see Methods) and refinement of single-crystal X-ray diffraction data (see Supplementary Fig. 1 ). Full size image The samples are air sensitive in powder form but visual inspection and magnetic measurements revealed no significant decay of larger single crystals on a timescale of hours. As stated in Gregory [30] , this is probably ‘due, somewhat perversely, to the formation of a surface film of predominantly LiOH’. Covering the samples with a thin layer of Apiezon M grease further protects the sample and no degradation was observed over a period of several weeks. Single crystals that had been exposed to air for a few minutes and were stored afterwards in an inert atmosphere (argon or nitrogen) did not change their magnetic properties on a timescale of 3 months. The electrical resistivity at room temperature is estimated to be ρ >10 5 Ω cm for all studied x . Magnetization Extreme magnetic anisotropy of Li 2 (Li 1– x Fe x )N is conspicuously evident in the magnetization measurements shown in Fig. 2a,b for two very different Fe concentrations of x =0.0032 and x =0.28. For magnetic field applied along the c axis, H ∥ c, the magnetization is constant for μ 0 H >1 T (starting from the field-cooled state) with a large saturated moment of per Fe atom. In contrast, the magnetization for H ⊥ c is smaller and slowly increases with field. A linear extrapolation to higher magnetic fields yields huge anisotropy fields of μ 0 H ani ≈88 T ( x =0.0032) and μ 0 H ani ≈220 T ( x =0.28) defined as the field strength where both magnetization curves intersect. The larger magnetic anisotropy field for x =0.28 is reflected in the larger coercivity field of μ 0 H c =11.6 T found for this concentration. The inverse magnetic susceptibility, χ −1 = H / M , roughly follows a Curie–Weiss behaviour for T ≳ 150 K and is strongly anisotropic over the whole investigated temperature range ( Fig. 2c ). The corresponding Weiss temperatures are and . In the following we discuss only measurements with H ∥ c since available laboratory fields do not allow saturation of the magnetization for H ⊥ c. Both and were found to be largely independent of the Fe concentration but for a small tendency to decrease with increasing x ( Fig. 1d , see Supplementary Note 4 for error analysis). The average values and are in good agreement with theoretical calculations for x =0.17 (ref. 24 ). Furthermore, the obtained effective moment is surprisingly close to the μ eff =6.6 μ B expectation value of a fully spin-orbit coupled state (Hund’s rule coupling), when assuming a 3 d 7 configuration for the proposed Fe +1 state (for a discussion of this unusual valence see refs 22 , 24 ). 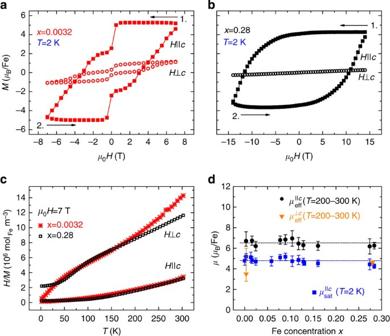Figure 2: Basic magnetic properties of Li2(Li1−xFex)N. (a,b) Large hysteresis in the magnetization,M(H), and a pronounced anisotropy depending on the orientation of the applied magnetic field,H, with respect to the crystallographic axes forx=0.0032 andx=0.28. WhereasMcan be saturated forH∥c, it is slowly increasing withHforH⊥cup to the highest available fields. (c) The temperature dependence of the inverse magnetization forx=0.28 follows a Curie–Weiss law forT≳150 K with effective moments offorH⊥candforH∥c. Similar behaviour is observed for the two orders of magnitude lower concentration ofx=0.0032, where the deviation forH⊥catT>200 K can be caused by a temperature-independent diamagnetic background of the Li3N host, which is negligible for higher Fe concentrations. (d) Bothμsatandμeffwere found to be largely independent ofxover the whole investigated range ofx=0.00028–0.28. The error bars are calculated based on the errors in assessing the sample mass and the Fe concentration and, forx=0.0032, on a diamagnetic contribution of the Li3N host. The average values areand. Figure 2: Basic magnetic properties of Li 2 (Li 1− x Fe x )N. ( a , b ) Large hysteresis in the magnetization, M(H) , and a pronounced anisotropy depending on the orientation of the applied magnetic field, H , with respect to the crystallographic axes for x =0.0032 and x =0.28. Whereas M can be saturated for H ∥ c, it is slowly increasing with H for H ⊥ c up to the highest available fields. ( c ) The temperature dependence of the inverse magnetization for x =0.28 follows a Curie–Weiss law for T ≳ 150 K with effective moments of for H ⊥ c and for H ∥ c . Similar behaviour is observed for the two orders of magnitude lower concentration of x =0.0032, where the deviation for H ⊥ c at T >200 K can be caused by a temperature-independent diamagnetic background of the Li 3 N host, which is negligible for higher Fe concentrations. ( d ) Both μ sat and μ eff were found to be largely independent of x over the whole investigated range of x =0.00028–0.28. The error bars are calculated based on the errors in assessing the sample mass and the Fe concentration and, for x =0.0032, on a diamagnetic contribution of the Li 3 N host. The average values are and . Full size image In the following, we focus on experimental results on the very dilute case that approaches an ideally non-interacting system of single magnetic atoms. The temperature dependence of the M - H loops for x =0.0032 with a high density of data points are shown in Fig. 3a . 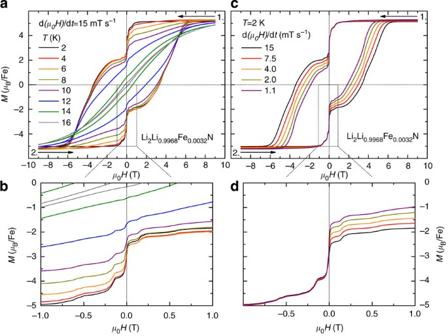Figure 3: Temperature and sweep rate dependence of the magnetization of Li2(Li1−xFex)N forx=0.0032,H∥c. (a) Hysteresis emerges forT≤16 K and the coercivity fields,Hc, are essentially temperature independent belowT=10 K. (b) The clear steps in the magnetization are smeared out with increasing temperature and disappear forT≳16 K. (c) The pronounced sweep rate dependence of the magnetization reveals the dynamic nature of the hysteresis. (d) Only the step atH=0 depends significantly on the sweep rate, indicating that the relaxation at the smaller steps atμ0H=±0.15 and ±0.55 T is fast on the timescale of the experiment. The step atH=0 is attributed to a flip of the Fe magnetic moment from below to above the crystallographica–bplane. The energy barrier associated with this transition seems to dominate the relaxation process and forms the global maximum in the magnetic anisotropy energy. The smaller steps are accordingly associated with tunnelling through smaller, local maxima. The following three main observations can be made: Figure 3: Temperature and sweep rate dependence of the magnetization of Li 2 (Li 1− x Fe x )N for x =0.0032, H ∥ c . ( a ) Hysteresis emerges for T ≤16 K and the coercivity fields, H c , are essentially temperature independent below T =10 K. ( b ) The clear steps in the magnetization are smeared out with increasing temperature and disappear for T ≳ 16 K. ( c ) The pronounced sweep rate dependence of the magnetization reveals the dynamic nature of the hysteresis. ( d ) Only the step at H =0 depends significantly on the sweep rate, indicating that the relaxation at the smaller steps at μ 0 H =±0.15 and ±0.55 T is fast on the timescale of the experiment. The step at H =0 is attributed to a flip of the Fe magnetic moment from below to above the crystallographic a–b plane. The energy barrier associated with this transition seems to dominate the relaxation process and forms the global maximum in the magnetic anisotropy energy. The smaller steps are accordingly associated with tunnelling through smaller, local maxima. Full size image First, the magnetization curve is essentially temperature independent for T <10 K with μ 0 H c =3.4 T, which indicates the irrelevance of thermal excitations. In contrast, H c changes dramatically between 10 and 16 K, indicating a distinct separation into a low- and a high-temperature behaviour. Second, there are pronounced steps in the magnetization. An enlarged view on part of the M - H loop, Fig. 3b , reveals steps in M at μ 0 H =0, ±0.15 and ±0.55 T. Another, smaller but well defined, step occurs at μ 0 H =±5 T. The step sizes are larger when H approaches zero and decrease with increasing temperature in contrast to the step positions, which are independent of temperature. No steps could be resolved for T ≳ 16 K. The steps are strongly suppressed with increasing x ( Supplementary Fig. 3 ), most likely caused by an increasing Fe–Fe interaction and vanish for x =0.28 ( Fig. 2b ). Third, the M - H loop at T =2 K starts from a saturated state where the Fe magnetic moments appear to be aligned parallel to the field, μ ∥ H with H ∥ c. The first step occurs already in the first quadrant (upper right corner) when H approaches zero from positive values. Similar behaviour was observed in lanthanide-based mononuclear SMMs [15] , whereas SMMs based on clusters show no corresponding steps in the first quadrant [1] . A decrease of the magnetization in the first quadrant, where H is still parallel to the initial magnetization, is incompatible with the c axis being the easy axis. Rather, the moment seems to be tilted away from the c axis and the reduced magnetization is the projection of the moment along the c axis (see Discussion). Notice that an axis canted away from the c axis would be 12- or 24-fold degenerate (depending on whether it is oriented along a high-symmetry direction like h 0 l or not). Accordingly, the magnetization perpendicular to the c axis ( H ⊥ c, M ⊥ c) is still small in zero field because the perpendicular components of the tilted moments cancel out. In contrast to a common ferromagnet, the M - H loops not only depend on temperature but also show a pronounced, characteristic dependence on the sweep rate of the applied magnetic field. Figure 3c,d shows M - H loops at T =2 K for sweep rates between 15 and 1.1 mT s −1 , corresponding to a total time between 40 min, and 9 h and 10 min, respectively, for the whole loop. The step sizes at μ 0 H =±0.15 and ±0.55 T hardly depend on the sweep rate, whereas the step size at H =0 does. A low sweep rate dependence of the step size is in accordance with a large tunnelling gap, which is much smaller than the energy gap [31] (for a convenient description of the relation between sweep rate and tunnelling gap see, for example, Wernsdorfer and Sessoli [32] and references therein). Although the field values for the steps do not change significantly with sweep rate, the width of the whole hysteresis loop (and therefore H c ) does ( Fig. 3c ). Pronounced sweep rate dependence of H c is observed also for higher Fe concentrations—see Supplementary Fig. 3 . The observation of smaller H c values in slower measurements clearly reveals the dynamic nature of the hysteresis. This observation motivated a detailed study of the time dependence of the magnetization, which is presented in the following section. Relaxation When a magnetic moment is subject to a change in the applied magnetic field, it will take a finite relaxation time to reach the equilibrium state (see, for example, Cullity [33] ). The sweep rate dependence of the hysteresis loops indicates a timescale of several hours for the relaxation in Li 2 (Li 1– x Fe x )N. This is so slow that the change of the magnetization with time, M ( t ), during the relaxation process can be directly measured by standard laboratory magnetometers. Three procedures are schematically shown in the left panels of Fig. 4 (see Supplementary Note 4 for detailed measurement protocols). The corresponding experimental data are in the panels to the right. 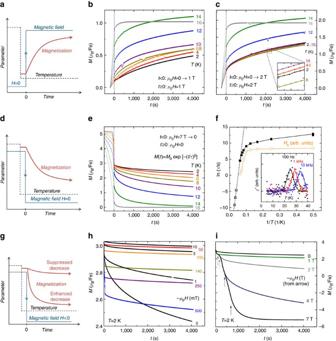Figure 4: Time dependence of the magnetization. (a,d,g) Schematics of different relaxation processes and corresponding experimental data on Li2(Li0.9968Fe0.0032)N to the right. (b) The increase in the magnetization as a function of time,M(t), belowT=10 K is only weakly temperature dependent forμ0H=1 T. (c) Increasing the applied field toμ0H=2 T leads to an essentially temperature-independent relaxation belowT=10 K, which is inconsistent with a thermally activated relaxation process. (e) Decrease inM(t)after ramping the field fromμ0H=7 T to 0.M(t)is fit to a stretched exponential function and the obtained relaxation times,τ, are shown as closed squares in the form of an Arrhenius plot in (f). (f)τdetermined from the imaginary part of the alternating current magnetic susceptibility,χ''(T) (inset), is shown by open squares. Thermally activated behaviour is observed at higher temperatures (dashed line). The formation of a plateau towards lower temperatures is incompatible with thermally activated behaviour and indicates the relevance of quantum tunnelling. The coercivity field (open circles, sweep rate 15 mT s−1) shows similar temperature dependence, indicating slow relaxation as the origin of spontaneous magnetization. (g) Small negative fields of a few milliTesla, applied opposite to the initial applied field ofμ0H=7 T, significantly reduce the decrease inM(t)compared withH=0. (i) In contrast,M(t)decreases faster in larger negative fields of |μ0H|≥1 T. Figure 4: Time dependence of the magnetization. ( a , d , g ) Schematics of different relaxation processes and corresponding experimental data on Li 2 (Li 0.9968 Fe 0.0032 )N to the right. ( b ) The increase in the magnetization as a function of time, M(t) , below T =10 K is only weakly temperature dependent for μ 0 H =1 T. ( c ) Increasing the applied field to μ 0 H =2 T leads to an essentially temperature-independent relaxation below T =10 K, which is inconsistent with a thermally activated relaxation process. ( e ) Decrease in M(t) after ramping the field from μ 0 H =7 T to 0. M(t) is fit to a stretched exponential function and the obtained relaxation times, τ , are shown as closed squares in the form of an Arrhenius plot in ( f ). ( f ) τ determined from the imaginary part of the alternating current magnetic susceptibility, χ'' ( T ) (inset), is shown by open squares. Thermally activated behaviour is observed at higher temperatures (dashed line). The formation of a plateau towards lower temperatures is incompatible with thermally activated behaviour and indicates the relevance of quantum tunnelling. The coercivity field (open circles, sweep rate 15 mT s −1 ) shows similar temperature dependence, indicating slow relaxation as the origin of spontaneous magnetization. ( g ) Small negative fields of a few milliTesla, applied opposite to the initial applied field of μ 0 H =7 T, significantly reduce the decrease in M(t) compared with H =0. ( i ) In contrast, M(t) decreases faster in larger negative fields of | μ 0 H |≥1 T. Full size image Figure 4a–c shows the relaxation after switching-on the field. M ( t ) increases rapidly for T =16 K and the magnetization is constant after t ~500 s. The relaxation is becoming markedly slower as the measurement temperature is reduced to T =10 K, and M ( t ) keeps increasing up to the maximum measurement time. However, below 10 K, M ( t ) is only weakly temperature dependent in μ 0 =1 T and essentially temperature independent in μ 0 H =2 T. This temperature independence is inconsistent with a thermally activated relaxation process. The inset of Fig. 4c shows an enlarged region of the plot. No correlation of relaxation with temperature is apparent. The relaxation for T >16 K is too fast to be measured directly and M ( t ) becomes immediately constant once the field is stabilized. The relaxation process shows clear anomalies at the resonance fields (step positions in M - H loops) as shown in Supplementary Fig. 4 . Figure 4d–f shows the relaxation after switching-off the field. The relaxation is fast for T =16 K but suppressed for lower temperatures. However, the decrease is non-uniform with temperature and markedly smaller at the lowest temperatures. M ( t ) can be fitted to a stretched exponential with M 0 = M ( t =0) and τ is the relaxation time (for details regarding the exponent β see Supplementary Fig. 5 and Supplementary Note 4 ). For T >16 K, τ is too small to be measured directly but can be determined from the out-of-phase part of the alternating current magnetic susceptibility, χ ′′( T ). The inset in Fig. 4f shows maxima in χ ′′( T ) at temperatures T max , which increase with the excitation frequency f . The maximum in χ ′′( T ) corresponds to a maximum in the energy absorption of the alternating magnetic field by the sample and shows that the relaxation time equals the timescale of the experiment, that is, τ =1/ f at T = T max . The values obtained for τ are shown in Fig. 4f in the form of an Arrhenius plot. For T ≥16 K, τ follows a linear (Arrhenius) behaviour with good agreement between directly and indirectly measured values. A fit of τ to a thermally activated law ( τ = τ 0 exp[Δ E / k B T ], dashed line) gives an energy barrier of Δ E / k B =430 K and a pre-exponential factor τ 0 =2.8 × 10 −10 s. For T <16 K, τ deviates significantly from Arrhenius behaviour and decreases much slower with decreasing temperature than expected for a thermally activated relaxation. A plateau, as shown in Fig. 4f , has been found in SMMs [2] , [34] and is a clear fingerprint of quantum tunnelling. Figure 4g–i shows the relaxation in negative fields. This method is a variation of the previous one where the field is not simply switched-off but ramped to a negative value opposite to the initial direction. As shown by the large magnetic hysteresis and the relaxation measurements above, the dominating energy scale of the system lies in the region of several Tesla acting on a few μ B . Therefore, a magnetic field of a few milliTesla can, at most, merely change the energy-level scheme. Furthermore, applying a negative field is expected to accelerate the decrease of M ( t ). In contrast to both assumptions, small fields of μ 0 H =−1 to −10 mT have a dramatic effect on the relaxation time and lead to an increase of τ by several orders of magnitude (black curves in Fig. 4h ). In fact, the relaxation in μ 0 H =−10 mT is becoming so slow that an accurate determination of τ is not possible within 4,000 s but requires much longer measurement times (which is beyond the scope of this publication). The main effect of the small negative field is likely a destruction of the tunnelling condition by lifting the zero-field degeneracy—resonant tunnelling of the magnetization occurs only between degenerate states [1] . In intermediate fields of μ 0 H =−50 to −500 mT, the magnetization decreases rapidly until the applied field is stable (that is, after 50 s for μ 0 H =−500 mT), followed by a significantly slower relaxation. This indicates the presence of two timescales for the relaxation, a fast one and a slow one. The slow relaxation can be associated with overcoming the large energy barrier in the a – b plane. However, the flipped moments are still not (anti-)parallel to the c axis ( Fig. 5a ). The fast relaxation can be associated with the subsequent, full alignment of the magnetic moments along the c axis by overcoming smaller, local maxima in the magnetic anisotropy energy (corresponding to the smaller steps in the M - H loop, see Fig. 5b ). Only larger fields of | μ 0 H |>1 T cause a faster decrease of M ( t ) when compared with zero field ( Fig. 4i ). A fast relaxation on the timescale of the experiment is reached at μ 0 H =−7 T where M ( t ) is saturated after t ≈2,000 s. Accordingly, the magnetization reaches saturation in a similar short time after applying a field of μ 0 H =7 T to an unmagnetized sample (analogue to Fig. 4a–c , not shown). It should be noted that the time dependencies, as presented in this section, are not restricted to low Fe concentrations. Clear relaxation effects are observed through the whole concentration range with the tendency to slow down with increasing x . 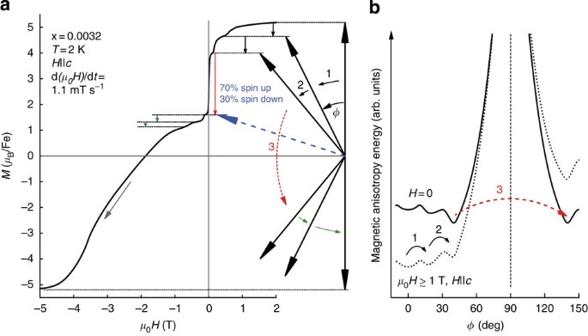Figure 5: Magnetic moment orientation and anisotropy energy. (a) Magnetization of Li2(Li1−xFex)N and a corresponding possible orientation of the magnetic moment. This simplified model assumes a constant magnitude of the magnetic moment independent of the orientation with respect to the c axis (ϕis the angle between moment and c axis). The plateau after step 2 corresponds toϕ~40°. The large jump inM(H) atH~0 is in accordance with a reorientation of 30% of the Fe magnetic moments from spin-up (ϕ~40°) to spin-down (ϕ~140°). A further rapid reorientation forH<0 is blocked because the resonance condition for magnetic tunnelling is destroyed forH≠0. (b) Possible schematic of the magnetic anisotropy energy as a function of the angle to the crystallographic c axis. The global minimum in zero field appears at an angle ofϕ~40°. Adding a sufficiently large Zeeman term for an applied field along the c axis (dotted line) leads to a global minimum located atϕ=0. The large step in theM-Hloop occurring at zero field is associated with the resonant tunnelling through the large energy barrier centred atϕ=90°. Accordingly, the smaller steps correspond to transitions from a local to the (actual) global minimum in the total magnetic energy. Figure 5: Magnetic moment orientation and anisotropy energy. ( a ) Magnetization of Li 2 (Li 1− x Fe x )N and a corresponding possible orientation of the magnetic moment. This simplified model assumes a constant magnitude of the magnetic moment independent of the orientation with respect to the c axis ( ϕ is the angle between moment and c axis). The plateau after step 2 corresponds to ϕ ~40°. The large jump in M ( H ) at H ~0 is in accordance with a reorientation of 30% of the Fe magnetic moments from spin-up ( ϕ ~40°) to spin-down ( ϕ ~140°). A further rapid reorientation for H <0 is blocked because the resonance condition for magnetic tunnelling is destroyed for H ≠0. ( b ) Possible schematic of the magnetic anisotropy energy as a function of the angle to the crystallographic c axis. The global minimum in zero field appears at an angle of ϕ ~40°. Adding a sufficiently large Zeeman term for an applied field along the c axis (dotted line) leads to a global minimum located at ϕ =0. The large step in the M - H loop occurring at zero field is associated with the resonant tunnelling through the large energy barrier centred at ϕ =90°. Accordingly, the smaller steps correspond to transitions from a local to the (actual) global minimum in the total magnetic energy. Full size image Our work shows that Li 2 (Li 1– x Fe x )N not only has a clear and remarkable anisotropy, generally not associated with Fe moments, but also shows time dependence more consistent with SMM systems. The strong correlation of relaxation time and coercivity field ( Fig. 4f ) indicates that the slow relaxation leads to magnetic hysteresis for x ≪ 1, that is, the dilute system is not a ferromagnet and hysteresis emerges from a slow decay of a polarized, paramagnetic state. Whether this holds true for the dense system ( x =0.28), too, is not settled at this point—below T ≈65 K the ordering appears to be static on the timescale of Mössbauer spectroscopy [22] , [23] (performed on polycrystalline material, x =0.16 and 0.21). A possible schematic for the magnetic moment orientation and the magnetic anisotropy energy is depicted in Fig. 5 . This model is purely based on the observed plateaus in the M - H measurements and, beyond the extreme uniaxial symmetry of the iron environment, the origin of the magnetic anisotropy of Li 2 (Li 1– x Fe x )N is still unclear. The anisotropy found in SMMs is based on the magnetic interactions within the transition metal cluster or in the single-ion anisotropy of lanthanide ions (or on both). For the latter case, the anisotropy is caused by the crystal electric field that acts as perturbation on the multiplet ground state of the lanthanide ion, which is determined by Hund’s rule coupling. Neither of these conceptionally simple scenarios is applicable for Li 2 (Li 1− x Fe x )N since the Fe atoms are too dilute to strongly interact with each other for x ≪ 1 and the crystal electric field is too strong to be regarded as a small perturbation when compared with the spin-orbit coupling. Instead we are left with the complex determination of the energy-level scheme of the relevant Fe-3 d electrons. Calculations based on LDA predict a counter-intuitive energy-level scheme with the 3 d z 2 level having the lowest energy followed by partially occupied , d xy levels [24] . A very similar energy-level scheme was recently found for a mononuclear Fe-based SMM [19] sharing a similar structural motif as the Fe site in Li 2 (Li 1− x Fe x )N: a linear Fe +1 complex, which seems to be an essential ingredient for the emergence of unquenched orbital moments and large magnetic anisotropy. Even though the exact microscopic origin of the energy barriers separating the magnetic states in Li 2 (Li 1− x Fe x )N is not yet understood, we argue that quantum tunnelling has to be invoked to overcome them. From the Arrhenius fit we find Δ/ k B =430 K ( Fig. 4f ). Magnetization measurements on single crystals allow for a second method to estimate the barrier height: when H reaches the anisotropy field, all moments are aligned along the field and the energy barrier is overcome. This gives rise to Δ E / k B ≈ μ 0 H ani × μ sat / k B ≈88T × 5 μ B / k B =300 K in reasonable agreement with the above result. This value also agrees with the LDA-based calculation of the anisotropy energy for x =0.17 (Δ/ k B =278 K) [24] . Such a large barrier cannot be overcome thermally at T =2 K—an estimation of the relaxation time from thermally activated law and Δ/ k B =278 K yields τ >10 43 years (give or take a millennium). Therefore, a tunnelling process is likely involved in the relaxation process where the applied magnetic field shifts the energy levels in and out of degeneracy in full analogy to SMMs. At this point it is not clear which levels of the single ion are brought in resonance by the applied magnetic field to explain the smaller steps in the M - H loops. Hyperfine interactions, as invoked for lanthanide-based SMMs [15] and LiY 0.998 Ho 0.002 F 4 (ref. 35 ), are probably too weak to account for steps at applied fields of μ 0 H =0.5 T in particular since 98% of the Fe atoms do not carry a nuclear moment. Energy barriers of similar (Δ/ k B =300 K [19] , [36] ) or even higher size (Δ/ k B =800 K [37] ) have been observed in mononuclear SMMs. However, the remanent magnetization for these samples is very small caused by short relaxation times at low temperatures, that is, τ deviates from Arrhenius behaviour with a relaxation time at the plateau in the order of seconds—in contrast to τ ~10 5 s found for Li 2 (Li 1− x Fe x )N. The fortunate combination of a deviation from Arrhenius behaviour at high temperatures ( T >10 K) with large values at the plateau leads to the extreme coercivities presented here. For potential data storage applications and stable magnetic materials, it is desirable to increase τ by suppressing the tunnel effect, which can be achieved by enhanced exchange coupling [11] , [38] . On the other hand, studying tunnelling phenomena by itself requires isolated magnetic moments. Both goals can be satisfied by varying the Fe concentration in Li 2 (Li 1− x Fe x )N accordingly. Thus for low Fe concentration of x =0.0032, statistically, 98% of the Fe atoms have only Li as the nearest neighbours in the a – b plane and Fe–Fe interactions are negligible. Larger Fe concentrations show higher coercivity fields at the lowest temperatures ( Supplementary Fig. 3 ), which are caused by larger relaxation times, indicating that Fe–Fe interactions are indeed detrimental to tunnelling. Provided the energy barriers can be further enhanced and tunnelling appropriately controlled, this opens a route for the creation of hard permanent magnets from cheap and abundant elements. One remaining question is: why is quantum tunnelling so elusive in inorganic compounds? Besides our discovery in Li 2 (Li 1− x Fe x )N, we are aware of only one other family of inorganic compounds showing macroscopic quantum tunnelling effects of the magnetization: LiY 0.998 Ho 0.002 F 4 (refs 26 , 35 ) and related systems. However, the characteristic energy scales are two orders of magnitude smaller than in Li 2 (Li 1− x Fe x )N and magnetic hysteresis emerges only below T =200 mK with coercivity fields of μ 0 H c =30 mT. To observe a macroscopic quantum effect such as tunnelling of the magnetization, the interaction between the magnetic moments has to be small. In general, coupling leads to excitations (modes), which lead to dissipation that destroys the quantum state. This rules out systems with dense, interacting moments. Diluted systems of local magnetic moments have been the subject of extensive research mainly to study the Kondo effect. This necessarily requires metallic samples; the magnetic moments are not isolated but coupled to the electron bath, which again leads to dissipation and the destruction of the quantum state. Insulating samples with diluted or non-interacting magnetic moments have been far less studied—diluted magnetic semiconductors are explicitly excluded from this statement because of their finite carrier density. A possible explanation for the absence of magnetic tunnelling in insulators is a Jahn–Teller distortion, which is frequently observed, for example, in lanthanide zircons of the form RXO 4 (Kirschbaum [39] and references therein). According to the Jahn–Teller theorem [40] , the orbital degeneracy of Fe should cause a structural distortion also for Li 2 (Li 1− x Fe x )N in order to reach a stable state. In the diluted case it will occur locally for Fe and not necessarily for the whole crystal. Lifting the orbital degeneracy corresponds to a zero-orbital angular momentum, which is the only fully non-degenerate state. Consequently, a Jahn–Teller distortion would lead to a loss of the magnetic anisotropy and a decay of the energy barrier. However, the Fe atom sits between two nitrogen neighbours, which provide the dominant bonding. These three atoms can be regarded as acting like a linear molecule, which is not subject to a Jahn–Teller distortion [40] . To summarize, we demonstrated a huge magnetic anisotropy and coercivity in Li 2 (Li 1− x Fe x )N and want to emphasize the three properties that are probably essential for the emergence of macroscopic quantum tunnelling: the compound is insulating, the orbital magnetic moment of Fe is not quenched and the N–Fe–N complex forms a linear molecule avoiding a Jahn–Teller distortion. These properties may serve as a basis for the design of materials featuring even higher characteristic energy scales. Crystal growth Starting materials were Li granules (Alfa Aesar, 99%), Li 3 N powder (Alfa Aesar, 99.4%) and Fe granules (99.98%). The mixtures had a molar ratio of Li:Fe:N=9− x 0 : x 0 :1 with x 0 =0–0.5. A total mass of roughly 1.5 g was packed into a 3-cap Ta crucible [41] inside an Ar-filled glovebox. The Ta crucible was sealed by arc melting under inert atmosphere of ~0.6 bar Ar and subsequently sealed in a silica ampoule. The Li–Fe–N mixture was heated from room temperature to T =900 °C over 4 h, cooled to T =750 °C within 1.5 h, slowly cooled to T =500 °C over 62 h and finally decanted to separate Li 2 (Li 1− x Fe x )N crystals from the excess liquid. Single crystals of hexagonal and plate-like habit with masses >100 mg could be obtained. The maximum lateral sizes of ≈10 mm were limited by the crucible size where the crystal thickness is typically ≈1 mm. Typically we found a few large single crystals with similar orientation clamped between the container walls above the bottom of the crucible and also several smaller ones attached to the bottom. We used pieces of the larger crystals for the magnetization measurements presented in this publication. It should be noted that the smallest Fe concentration of x =0.00028, as measured by ICP–MS (see below), was obtained without intentional introduction of Fe in the melt. Fe was most likely introduced as an impurity from the starting materials or from the Ta crucible. Chemical analysis with ICP–MS The Li 2 (Li 1− x Fe x )N samples were analysed using an inductively coupled plasma magnetic sector mass spectrometer (ICP–MS, Element 1, Thermo Scientific). The samples were introduced into the ICP via a low-flow nebulizer (PFA-100, Elemental Scientific Inc.) and double-pass spray chamber. The interface between the ICP and mass spectrometer was equipped with nickel sampler and skimmer (H-configuration) cones. The mass spectrometer was operated in medium resolution ( m /Δ m =4,000) to separate the Fe + isotopes of interest from interfering species. The detector was operated in dual mode, allowing for the operating software to selectively switch between analogue and counting measurements. Prior to sample analysis, the torch position and instrumental operating parameters ( Table 1 ) were adjusted for maximum peak height and signal stability. The main elements of interest for quantification were lithium (mass-to-charge ratio m / z =7) and iron ( m / z =55.935 and 56.935). Tantalum ( m / z =181) and calcium ( m / z =43 and 44) were also measured to check for contamination from the crucible material and known impurities of the starting materials. Following these initial analyses, a full isotopic spectrum ( m / z =7–238) was measured in low resolution ( m /Δ m =300) for several representative samples to check for any other possible sources of contamination. Carbon, nitrogen and oxygen could not be measured due to high background levels contributed by the acid solution, the argon gas and the instrumental components. Minor amounts of tantalum and calcium were measured in the Li–Fe–N samples. All samples contained less than 0.4 mass% calcium (corresponding to Li 1− δ Ca δ with δ <0.007) and less than 0.1 mass% tantalum (corresponding to Li 1− δ Ta δ with δ<0.0004). The combined concentrations of all other contaminant elements comprised far less than 0.01 mass% of the solid samples. Table 1 ICP–MS operating parameters. Full size table All of the Li 2 (Li 1− x Fe x )N samples were dissolved for ICP–MS analysis. Approximately 5–25 mg of solid sample was weighed accurately into an acid vapour-washed Teflon bottle on a balance. A small amount (2–4 g) of cold (~3 °C) deionized water was added and allowed to react. Once the sample mass stabilized, ~1.5 g of 70% nitric acid was added to completely dissolve the remaining solid. On complete dissolution, the solution was diluted with deionized water to a mass of 50 g. Aliquots of these original solutions were diluted with prepared aqueous 1% nitric acid to a concentration of 1–5 p.p.m. in terms of the original solid sample mass. Standard solutions were prepared for the quantification of iron and lithium in the samples. A 1 p.p.m. iron and lithium standard was prepared by diluting 1,000 p.p.m. stock solutions (SPEX CertiPrep, High-Purity Standards) with cleaned 1% nitric acid. Lower concentration standards were prepared via dilutions of the original 1 p.p.m. standard solution. Blanks of the water and acids were analysed and had negligible amounts of the analyte elements. The water used was 18 MΩ cm (Barnstead Nanopure) and the nitric acid was purified by sub-boiling distillation (Classic Sub-boiling Still Assembly, Savillex) before use. Lithium is prone to memory effects in ICP–MS due to either sample introduction or deposition and vaporization of Li from the cones. The Li + (and Fe + ) signals from the samples and standards all rinsed out to baseline between the measurements. How to cite this article: Jesche, A. et al. Giant magnetic anisotropy and tunnelling of the magnetization in Li 2 (Li 1− x Fe x )N. Nat. Commun. 5:3333 doi: 10.1038/ncomms4333 (2014).